Loss of Wdfy3 in mice alters cerebral cortical neurogenesis reflecting aspects of the autism pathology Autism spectrum disorders (ASDs) are complex and heterogeneous developmental disabilities affecting an ever-increasing number of children worldwide. The diverse manifestations and complex, largely genetic aetiology of ASDs pose a major challenge to the identification of unifying neuropathological features. Here we describe the neurodevelopmental defects in mice that carry deleterious alleles of the Wdfy3 gene, recently recognized as causative in ASDs. Loss of Wdfy3 leads to a regionally enlarged cerebral cortex resembling early brain overgrowth described in many children on the autism spectrum. In addition, affected mouse mutants display migration defects of cortical projection neurons, a recognized cause of epilepsy, which is significantly comorbid with autism. Our analysis of affected mouse mutants defines an important role for Wdfy3 in regulating neural progenitor divisions and neural migration in the developing brain. Furthermore, Wdfy3 is essential for cerebral expansion and functional organization while its loss-of-function results in pathological changes characteristic of ASDs. With a global median prevalence of 62 per 10,000 autism spectrum disorders (ASDs, used interchangeably with autism in this paper) are among the most common neurodevelopmental conditions [1] . ASDs typically become apparent after the second year of life and are characterized by a triad of behavioural deficits affecting reciprocal social interaction, language development, as well as interests and activities [2] . In recent years, a strong, albeit very heterogeneous, genetic component to the aetiology of ASDs has been recognized [3] , [4] , [5] , [6] , [7] . Estimates from these studies suggest that genes causative in the pathology of ASDs may number in the hundreds, and possibly up to a thousand, but may converge on just a few basic cellular pathways. For instance, several mutations were identified in genes encoding factors required for synaptic connectivity and signalling, thus highlighting functional defects at the chemical synapse as one physiological root cause of ASDs [8] , [9] , [10] . In addition, several independently replicated studies identified anomalies in brain development resulting in early brain overgrowth as a common feature in a subset of individuals with ASDs [11] , [12] , [13] . Recently, the cause of this overgrowth in the prefrontal cortex has been found to be centred on a long-suspected increase in projection neuron numbers [14] . Intriguingly, a current study described excess of neurons in autism to be also associated with patches of disrupted laminar organization of the cerebral cortex (Cx) [15] . As cerebral cortical neurogenesis and layer formation occurs exclusively during late embryonic and fetal development [16] , these studies provided strong evidence for a prenatal origin of many autism cases. This notion was further strengthened by the analysis of coexpression networks of known autism disease genes, which implicate midfetal deep layer projection neurons as a point of convergence for the autism pathology [17] . Two interesting features, whose significance and causes remain uncertain at this point, have been linked to early brain overgrowth-associated autism. First, brain enlargement is noticeable only in early childhood, typically plateaus around age seven and often regresses later in life compared with unaffected controls [11] , [12] , [13] . Second, size increases appear regionally restricted to frontal and temporal lobes while parietal and occipital lobes appear mostly unaffected [11] , [13] . Previous genome-wide linkage analysis identified an autism susceptibility locus at 4q with a peak between markers D4S2361 and D4S2909 (4q21.23-22.3) [18] . In addition, an autism case was described with a 16.5 Mbp deletion at 4q21.23-q24 (ref. 19 ). This region contains the WDFY3 gene, in which a de novo nonsense mutation was recently identified in a child on the autism spectrum from the Simons Simplex Collection [7] . Taken together, these results suggest that WDFY3 is a human disease gene that, if mutated, leads to autism. Interestingly, the sole known function of WDFY3 is to act as an adaptor protein by linking specific proteins destined for degradation to the core autophagic machinery in a process termed selective macroautophagy. WDFY3 is a member of the BEACH (beige and CHS proteins) protein family and contains in addition to the BEACH domain five WD40 domains and a C-terminal FYVE (Fab1/YOTB/Vac1/EEA1) domain [20] . WDFY3 has been shown to interact directly with the lipid membrane component phosphatidylinositol 3-phosphate through its FYVE domain [20] , with Atg5 through its WD40 repeats [21] , and with P62 through its BEACH domain [22] . However, the way in which WDFY3 influences typical brain development and how its loss-of-function may precipitate neurodevelopmental anomalies underlying ASDs remained unexplained and warranted closer examination. Through the analysis of two separate lines of Wdfy3 -deficient mice, one generated by random mutagenesis and one by gene targeting, we have identified an essential role for Wdfy3 in cerebral cortical histogenesis. Wdfy3 loss-of-function in our mouse models leads to both an increase in proliferative neural progenitor divisions resulting in an increase in cerebral cortical size as well as focal cortical dysplasias. Abnormal brain morphology in Wdfy3 -mutant mice In a forward genetic screen aimed at identifying mutations affecting forebrain development, we recovered a line of mice displaying loss of thalamocortical connectivity inherited in an autosomal recessive manner [23] . We named the line disconnected (disc) and, by positional mapping, restricted the mutation to a 2.46 Mbp interval on chromosome 5 containing 10 protein-coding genes ( Fig. 1a ). Sequencing of all coding sequences, splice sites and an average of 50 bp of adjacent introns of the genes within the interval identified a single nonsense mutation in exon 59 of 67 of the Wdfy3 gene (T to A at position 9,683 of NM_172882, aa 3,046 of 3,508; Fig. 1b,c ). Wdfy3 has been characterized as a crucial component of the autophagy pathway for mediating the selective autophagic degradation of macromolecular components such as aggregation-prone proteins [20] , [21] , [22] . Homozygote disc mutants die perinatally for unknown reasons while heterozygotes show no overt neurodevelopmental anomalies, have a normal lifespan and are fertile. 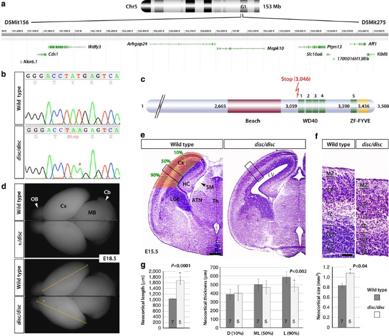Figure 1: Positional mapping of thediscallele and forebrain overgrowth in homozygous mutants. (a) The diagram shows the genomic interval on chromosome 5 between markers D5Mit156 and D5Mit275 to which thediscmutation was mapped. All protein-encoding genes within the interval of which all exons were sequenced for this study are shown. (b) Sequence chromatograms of WT anddisc/discPCR amplicons show the position of the only identified coding variant (T to A, nonsense). (c) The schematic shows the recognized domains of mouse Wdfy3 protein with the causative stop codon of thediscallele at position 3,046 indicated. The first residue of each domain is given in the diagram. (d) Dorsal views of whole-mount brains show morphological anomalies in the homozygousdiscmutants where indicated by the asterisk. (e) Nissl-stained coronal hemisections through the forebrains of E15.5 WT and homozygousdiscmutants illustrate the malformations present in affected mutants. The green lines delineate the measurements taken for cortical length and thickness (D, dorsal; ML, mediolateral; L, lateral), while the orange area indicates how cortical size was measured. (f) Close-ups of the mediolateral Cx illustrate cortical thinning indisc/discmutants. (g) Quantification of individual cortical spatial parameters confirm significant increases in length and overall size, but radial thinning in basolateral aspects. All analysis by Student’st-test,nfor either genotype is indicated in the bar diagrams, which present mean and s.e.m. Asterisks mark significant changes with calculatedPvalues shown. ATN, anterior thalamic nuclei; Cb, cerebellum; CP; HC, hippocampus; IZ, intermediate zone; LGE, lateral ganglionic eminence; LV, lateral ventricles; MZ, marginal zone; SM, stria medullaris; SVZ, subventricular zone; Th, thalamus; VZ, ventricular zone. Scale bar ineis 500 μm and inf100 μm. Figure 1: Positional mapping of the disc allele and forebrain overgrowth in homozygous mutants. ( a ) The diagram shows the genomic interval on chromosome 5 between markers D5Mit156 and D5Mit275 to which the disc mutation was mapped. All protein-encoding genes within the interval of which all exons were sequenced for this study are shown. ( b ) Sequence chromatograms of WT and disc/disc PCR amplicons show the position of the only identified coding variant (T to A, nonsense). ( c ) The schematic shows the recognized domains of mouse Wdfy3 protein with the causative stop codon of the disc allele at position 3,046 indicated. The first residue of each domain is given in the diagram. ( d ) Dorsal views of whole-mount brains show morphological anomalies in the homozygous disc mutants where indicated by the asterisk. ( e ) Nissl-stained coronal hemisections through the forebrains of E15.5 WT and homozygous disc mutants illustrate the malformations present in affected mutants. The green lines delineate the measurements taken for cortical length and thickness (D, dorsal; ML, mediolateral; L, lateral), while the orange area indicates how cortical size was measured. ( f ) Close-ups of the mediolateral Cx illustrate cortical thinning in disc/disc mutants. ( g ) Quantification of individual cortical spatial parameters confirm significant increases in length and overall size, but radial thinning in basolateral aspects. All analysis by Student’s t -test, n for either genotype is indicated in the bar diagrams, which present mean and s.e.m. Asterisks mark significant changes with calculated P values shown. ATN, anterior thalamic nuclei; Cb, cerebellum; CP; HC, hippocampus; IZ, intermediate zone; LGE, lateral ganglionic eminence; LV, lateral ventricles; MZ, marginal zone; SM, stria medullaris; SVZ, subventricular zone; Th, thalamus; VZ, ventricular zone. Scale bar in e is 500 μm and in f 100 μm. Full size image First, we examined forebrain morphology and focused our attention on the Cx. Analysis of the whole-mount mutant brains at embryonic day (E) 18.5 revealed no overt changes in disc heterozygotes compared with wild type (WT); however, homozygous mutants showed a characteristic enlargement of the most frontal aspects of the cortex accompanied by a reduction in the size of the olfactory bulbs ( Fig. 1d ; Supplementary Fig. 1 ). We then expanded our analysis of morphological changes in affected disc mutants by examining Nissl-stained coronal sections of various developmental stages. Our analysis revealed that, starting as early as E11.5, the forebrain of disc/disc mutants shows overt neurodevelopmental anomalies affecting the ganglionic eminences, which appear with a less rounded outline, while the ventricles are enlarged ( Supplementary Fig. 2 ). These anomalies continue to persist at later stages, during which also the Cx of homozygous disc mutants appears affected, by being visibly thinner and tangentially longer compared with WT controls ( Fig. 1e–g ). By taking measurements of individual morphological parameters of cortical sections during a period of peak neurogenesis (E15.5), we identified the most striking change to be a significant 62% increase in mutant neocortical length (Student’s t -test, P <0.001, WT n =7, disc/disc n =5; Fig. 1e,g ). Interestingly, neocortical thinning was not uniform along the dorsoventral axis of the neocortex but gradually decreased towards dorsal positions and was only significant at the most lateral measurement site (L) where the disc/disc neocortex was reduced by ~20% compared with WT (Student’s t -test, P <0.01) ( Fig. 1e,g ). Closer examination of cortical segments revealed that the proliferative regions of the ventricular and subventricular zones (VZ, SVZ) as well as the intermediate zone (IZ) were thinner in disc/disc mutants, while the cortical plate and marginal zone were not affected in thickness at this stage in development ( Fig. 1f ). With the combined effects of the lengthening and thinning of the neocortex, the total neocortical area is significantly enlarged in the disc/disc mutants by about 30% (Student’s t -test, P <0.02). As cortical measurements excluded any extracortical space, and in particular ventricular space, any cortical area increase in the disc/disc mutants does not reflect ventricular enlargement in these mice. These phenotypic changes are fully penetrant, observed throughout prenatal development and are of no tangible variability on different genetic backgrounds. In contrast, heterozygous disc mutants do not show any of these neurodevelopmental anomalies and appear phenotypically WT ( Supplementary Fig. 1 ). In summary, our findings demonstrate a tangential expansion but lateral thinning of the neocortical neuroepithelium, potentially pointing towards an imbalance in the mode of cortical progenitor cell divisions favouring proliferative over differentiative divisions, as previously shown in more severely affected mutant mouse models [24] , [25] . Furthermore, our findings of anterolateral regional enlargement appear consistent with several reports of transient megalencephaly in autism predominantly affecting frontal and temporal cerebral aspects [26] , [27] , [28] , [29] , [30] . Wdfy3 regulates the proliferation of neural progenitors Since morphological analysis suggested a proliferative shift of progenitor divisions in the disc/disc -mutant brains, we decided to assess the number of Pax6 + cortical radial glia cells [31] in the disc/disc mutant and compare it with the WT. In the developing cortex, the cells predominantly generated through symmetric proliferative divisions are radial glia and a shift towards such divisions should increase the Pax6 + radial glia population. Indeed, by measuring the area of Pax6 + cells along the cortical VZ of the disc/disc mutant, we found it to be significantly increased compared with the WT at stages E12.5 and E14.5 (Student’s t -test, P <0.04 and P <0.05 respectively, n =3 either genotype and stage; Fig. 2a,b ). No changes were detected in the density of Pax6 + cells within the VZ ( Fig. 2c,d ). Interestingly, a thinning of the Pax6 + VZ was observed at E14.5 at the most lateral positions consistent with the previous morphological analysis. Taken together, these data demonstrate that the functional loss of Wdfy3 results in an increase in the proliferation of Pax6 + radial glia at the neocortical VZ. 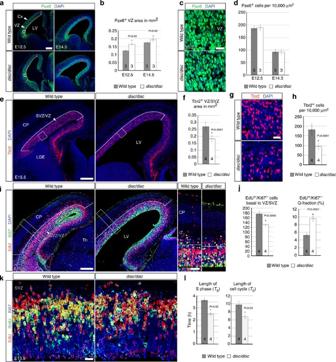Figure 2: Neural progenitor proliferation and neurogenesis are altered in homozygousdisc/discembryos. (a) Immunofluorescent analysis of Pax6 expression in the neocortical neuroepithelium at E12.5 and E14.5. Yellow dashed lines in the E12.5 brains outline the measured area of the Pax6+VZ. Red lines at E14.5 highlight the lateral thinning of the VZ. (b) Quantification of the Pax6+VZ reveals significant increases in thedisc/discmutant for either stage. In contrast, density of Pax6+cells is not altered in thedisc/discembryos (c,d). (e–h) Immunofluorescent area and density analysis of Tbr2+intermediate progenitors reveal significant reductions in both domains. (i,j) A 24 h EdU pulse-chase assay reveals a reduction in total neuronal output (EdU+/Ki67−cells basal to the SVZ) per hemisphere but an increase in the Q-fraction of cells that have exited the cell cycle. (k) Representative coronal sections of mediolateral cortex illustrate the outcome of time-shifted dual thymidine-labelling experiment and the distribution of EdU-, BrdU- and Ki67-labelled cells at E13.5. (l) Quantification of S-phase length (TS) and total cell cycle length (TC) determined significant decreases in thedisc/discmutants relative to WT. All statistical analysis by Student’st-test. Bar diagrams show mean and s.e.m., indicatenfor either genotype and calculatedPvalues of significant changes (asterisks). CP; Cx; IZ, intermediate zone; LV, lateral ventricles; Th, thalamus. Scale bar inais 200 μm, inc10 μm, ine100 μm, ing20 μm, ini100 μm and 50 μm, and ink20 μm. Figure 2: Neural progenitor proliferation and neurogenesis are altered in homozygous disc/disc embryos. ( a ) Immunofluorescent analysis of Pax6 expression in the neocortical neuroepithelium at E12.5 and E14.5. Yellow dashed lines in the E12.5 brains outline the measured area of the Pax6 + VZ. Red lines at E14.5 highlight the lateral thinning of the VZ. ( b ) Quantification of the Pax6 + VZ reveals significant increases in the disc/disc mutant for either stage. In contrast, density of Pax6 + cells is not altered in the disc/disc embryos ( c , d ). ( e – h ) Immunofluorescent area and density analysis of Tbr2 + intermediate progenitors reveal significant reductions in both domains. ( i , j ) A 24 h EdU pulse-chase assay reveals a reduction in total neuronal output (EdU + /Ki67 − cells basal to the SVZ) per hemisphere but an increase in the Q-fraction of cells that have exited the cell cycle. ( k ) Representative coronal sections of mediolateral cortex illustrate the outcome of time-shifted dual thymidine-labelling experiment and the distribution of EdU-, BrdU- and Ki67-labelled cells at E13.5. ( l ) Quantification of S-phase length ( T S ) and total cell cycle length ( T C ) determined significant decreases in the disc/disc mutants relative to WT. All statistical analysis by Student’s t -test. Bar diagrams show mean and s.e.m., indicate n for either genotype and calculated P values of significant changes (asterisks). CP; Cx; IZ, intermediate zone; LV, lateral ventricles; Th, thalamus. Scale bar in a is 200 μm, in c 10 μm, in e 100 μm, in g 20 μm, in i 100 μm and 50 μm, and in k 20 μm. Full size image An increase in proliferative divisions of radial glia in disc/disc embryos may occur on the expense of differentiative divisions, negatively affecting the number of Tbr2 + intermediate progenitors, which are predominantly generated through differentiating symmetric divisions of radial glia cells [31] , [32] , [33] . To follow up on this question, we assessed the number of intermediate progenitors by analysing the extent of the Tbr2 + area and density of Tbr2 + cells at E15.5. Indeed, our analysis confirmed significant reductions in both domains in the disc/disc mutants (Student’s t -test, P <0.0001 for area and density, n =4 either genotype). Specifically, we found the Tbr2 + area encompassing the VZ and SVZ to be reduced by ~30% and density of Tbr2 + cells to be reduced by ~50% ( Fig. 2e–h ). This finding provides further support for the concept that the increase of proliferative divisions in homozygous disc embryos may occur on the expense of differentiating divisions producing intermediate progenitors. As changes in proliferation dynamics of the disc/disc mutants will likely have consequences for developmental neurogenesis, we also assessed the number of postmitotic cells generated at E15.5 near the peak period of neurogenesis in the mouse. To that effect, we employed a 24 h thymidine-labelling approach using 5-ethynyl-2′-deoxyuridine (EdU). To take into consideration the regional differences in cortical malformation present in the disc/disc embryos, we counted all EdU + cells that had migrated basal to the SVZ within an entire hemisphere. To label and exclude cells still undergoing division, we used the proliferation marker Ki67. Using this approach, we identified a significant reduction of ~25% in EdU + /Ki67 − cells in the disc/disc mutants (Student’s t -test, P <0.0005, n =4 either genotype), largely driven by loss of postmitotic cells in the thinner basolateral cortical aspects ( Fig. 2i,j ). Interestingly, assessing in 200 μm wide cortical segments the quit (Q)-fraction of cells that had exited the cell cycle, we found it to be significantly increased by ~20% in the disc/disc embryos (Student’s t -test, n =4 either genotype, P <0.0005; Fig. 2i,j ). This finding likely points towards a more rapid turnover of intermediate progenitors into neurons, despite the overall reduced number of Tbr2 + cells. A central role has been recognized in the duration of the cell cycle of cortical neural progenitors for the sequential generation of neurons, as cell cycle length increases from inner to outer layer neuron production. In the mouse, this leads to more than doubling of cell cycle length during the course of cerebral cortical neurogenesis between E11 and E17, largely driven by an increase in G1 phase [34] . Furthermore, multiple studies have connected cell cycle length to the mode of progenitor divisions [35] , [36] , [37] , [38] , [39] . As our data supported the concept of changes in the mode of neural progenitor divisions in disc/disc mutants, we investigated whether these changes are also associated with altered cell cycle kinetics in affected disc mutants compared with the WT. To examine cell cycle progression in neural progenitors, we opted for a dual thymidine labelling approach following previously established paradigms [40] , [41] . Specifically, we injected pregnant mice with EdU followed 1.5 h later by an injection with 5-bromo-2′-deoxyuridine (BrdU) and sacrificed the embryos 30 min thereafter. As a result, cells which remained throughout the duration of the experiment in S phase were labelled with EdU and BrdU, while cells which exited S phase before BrdU exposure were labelled with EdU only. Cells that entered S phase at the end of the experiment were labelled predominantly with BrdU. The duration of the experiment ( T I ) was divided by ratios of single over double-labelled cells to generate estimates of S-phase length ( T S ) and total cell cycle length ( T C ). Analysing cortical segments in this manner, we found the length of T S to be significantly decreased from ~3.6 h in the WT to 2.5 h in the disc/disc mutants at E13.5 (Student’s t -test, P <0.02, n =4 either genotype; Fig. 2k,l ). Correspondingly, T C was found significantly decreased from ~9.8 h in the WT to 6.8 h in the disc/disc mutants confirming a more rapid mode of progenitor divisions in affected mutants. To further explore the idea that Wdfy3 regulates the proliferation of cortical progenitor cells, we next examined the developmental distribution of Wdfy3 using both RNA in situ hybridization and immunofluorescence analysis. RNA in situ hybridization analysis at E13.5 revealed highest Wdfy3 expression within the proliferative regions surrounding the ventricles ( Supplementary Fig. 3a ). Immunofluorescent analysis shows specific expression in the leptomeninges, cortical intermediate zone, choroid plexus and clusters of cells within the VZ ( Supplementary Fig. 3b ). On closer examination of the VZ, Wdfy3 expression is observed in a subset of cells actively undergoing mitosis ( Fig. 3a ). Wdfy3 expression persists through all phases of cell division, but becomes decreased during telophase. Wdfy3 expression is often maintained in radial units (possibly clones), which include also nondividing cells, and are projecting into the SVZ. Within these radial units, Wdfy3 expression appears highest in progenitors closest to the ventricle then gradually diminishes as distance from the ventricular surface increases. In nondividing cells, Wdfy3 localization appears largely cytosolic with possible perinuclear enrichment and presence in the glial endfeet. Moreover, co-labelling with Pax6, a marker for cortical radial glia, revealed that all Wdfy3 + cells in the VZ are radial glia cells, while Tbr2 + intermediate progenitors of the SVZ do not express Wdfy3 ( Fig. 3b ). Wdfy3 + cells present only a subset of dividing progenitors and are surrounded by Wdfy3 − mitotic cells. To further evaluate whether the loss of Wdfy3 function in the disc/disc embryos had an effect on cellular proliferation within the VZ, we analysed the number of phospho-histone H3 + mitotic cells that were also Wdfy3 + and compared them with the WT at stages E12.5 and E14.5 ( Fig. 3c,d ). For both stages, we found a significant reduction in the percentage of Wdfy3 + mitotic cells in the mutant (Student’s t -test, P <0.004 and P <0.0003, respectively, n =4 either genotype and stage) further supporting the notion that Wdfy3 is required for a specific subset of progenitor divisions and its loss-of-function will impair Wdfy3 + mitoses. To test whether loss of Wdfy3 may also result in loss of cells through cell death, we assessed the number of apoptotic cells by employing a terminal deoxynucleotidyl transferase dUTP nick-end labelling assay. By counting terminal deoxynucleotidyl transferase dUTP nick-end labelling positive + apoptotic cells throughout the entire cortical hemispheres, we see no significant differences between WT and disc/disc embryos (Student’s t -test; Supplementary Fig. 4 ), further confirming that cell loss is not a contributing factor to the morphological anomalies present in the Wdfy3-deficient cortex. 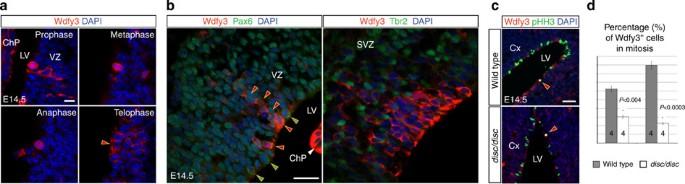Figure 3: Wdfy3 is upregulated in a subset of radial glia divisions during neurogenesis. (a) Immunofluorescent detection of Wdfy3 in cortical neural progenitors positioned at the ventricle of the WT cerebral cortex at E14.5 illustrates upregulation in dividing cells throughout all stages of mitosis. (b) Wdfy3 coexpression analysis with Pax6, a marker of radial glia and Tbr2, a marker of intermediate progenitor. Wdfy3+cells present only a subset of dividing progenitors (red arrowheads) and are surrounded by Wdfy3−mitotic cells. (c) Coexpression analysis of Wdfy3 with the mitosis marker phospho-histone H3+(pHH3) confirms that only a small share of mitotic cells is Wdfy3+. (d) Quantification of Wdfy3+/pHH3+cells at E12.5 and E14.5 shows significant reductions in thedisc/discmutants. Analysis by Student’st-test. Bar diagrams show mean and s.e.m., number of analysed embryos (n) and calculatedPvalues are indicated in the diagrams. Scale bar inais 10 μm, inb20 μm and inc40 μm. Figure 3: Wdfy3 is upregulated in a subset of radial glia divisions during neurogenesis. ( a ) Immunofluorescent detection of Wdfy3 in cortical neural progenitors positioned at the ventricle of the WT cerebral cortex at E14.5 illustrates upregulation in dividing cells throughout all stages of mitosis. ( b ) Wdfy3 coexpression analysis with Pax6, a marker of radial glia and Tbr2, a marker of intermediate progenitor. Wdfy3 + cells present only a subset of dividing progenitors (red arrowheads) and are surrounded by Wdfy3 − mitotic cells. ( c ) Coexpression analysis of Wdfy3 with the mitosis marker phospho-histone H3 + (pHH3) confirms that only a small share of mitotic cells is Wdfy3 + . ( d ) Quantification of Wdfy3 + /pHH3 + cells at E12.5 and E14.5 shows significant reductions in the disc/disc mutants. Analysis by Student’s t -test. Bar diagrams show mean and s.e.m., number of analysed embryos ( n ) and calculated P values are indicated in the diagrams. Scale bar in a is 10 μm, in b 20 μm and in c 40 μm. Full size image To examine in greater detail the characteristics of the cortical dysplasia in the disc/disc mice, we next analysed the distribution of the cortical layer-specific markers Tbr1 (layer 6) and Ctip2 (layer 5) at postnatal day (P) 0 to determine if any defects in radial migration or cortical lamination were present. Our analysis revealed that exclusively within the somatosensory area of the disc/disc -mutant neocortex heterotopic clusters of cells migrate to superficial laminar positions forming focal cortical dysplasia ( Fig. 4 ). Most heterotopia are comprised of only a few dozen cells with limited radial dispersion suggesting a possible origin from Wdfy3 + clusters undergoing pathological changes in disc/disc mutants. Interestingly, multifocal neocortical dysplasias are also a described feature of the autism pathology and underlying cause of epilepsy, which shows strong comorbidity to autism [15] , [42] . 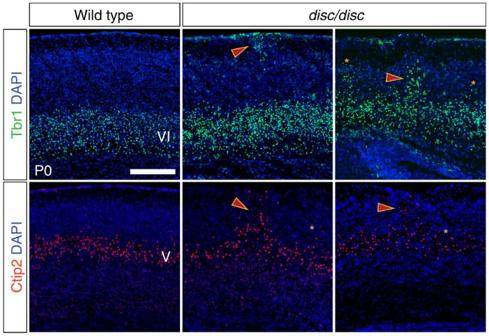Figure 4: Homozygousdiscmutants exhibit neuronal migration defects. Immunofluorescent analysis of cortical lamination markers Tbr1 (layer VI) and Ctip2 (layer V) reveals abnormalities in layer formation ofdisc/discmutants at P0. Arrowheads point to individual focal heterotopia of displaced cells for either marker in the mutant. Asterisks highlight smaller scale lamination anomalies. All sections shown are in the coronal plane of the somatosensory cortex. Scale bar, 200 μm. Figure 4: Homozygous disc mutants exhibit neuronal migration defects. Immunofluorescent analysis of cortical lamination markers Tbr1 (layer VI) and Ctip2 (layer V) reveals abnormalities in layer formation of disc/disc mutants at P0. Arrowheads point to individual focal heterotopia of displaced cells for either marker in the mutant. Asterisks highlight smaller scale lamination anomalies. All sections shown are in the coronal plane of the somatosensory cortex. Scale bar, 200 μm. Full size image Abnormal brain morphology in transgenic Wdfy3 mutants While the homozygous disc mice demonstrate several interesting characteristics of commonly described human ASD-like neuroanatomical defects, the animals die at birth while heterozygous disc carriers do not display any overt neurodevelopmental alterations, thus imposing limitations on utilizing this line as a suitable autism model. To further facilitate our analysis of Wdfy3 function in neural development and possibly create a more suitable model of human disease, we developed a series of alternative Wdfy3 alleles ( Wdfy3 lacZ , Wdfy3 loxP ) using targeted mutagenesis in collaboration with the Knockout Mouse Project and Mouse Biology Program at UC Davis ( Supplementary Fig. 5 ). Comparable to homozygous disc mutants, homozygous lacZ mice die perinatally for unknown reasons while lacZ heterozygotes have a normal lifespan and are fertile. Morphological analysis of brains of +/lacZ and lacZ/lacZ newborn pups revealed similar but more severe phenotypic changes compared with +/disc and disc/disc mice, respectively ( Fig. 5a–c ). The lacZ/lacZ brains show an even more drastic thinning and lengthening of the neocortex compared with homozygous disc mutants. We measured the overall cerebral size increase of the lacZ/lacZ brains to be ~13% (Student’s t -test, P <0.02, WT n =5, lacZ/lacZ n =4). Similar to the disc/disc mice, the lacZ/lacZ mutants exhibit a significant 16% reduction in cortical thickness only in the most lateral position (Student’s t -test, P <0.02 in comparison with WT), but an observable trend towards thinning throughout the cortex. However, unlike the +/ disc mice, the +/lacZ mice display a mild, but significant increase in the cortical length of ~19% (Student’s t -test, P <0.04, WT n =5, + /lacZ n =8). This cortical lengthening, however, does not result in a significant overall cortical size increase in +/lacZ mutants (Student’s t -test). 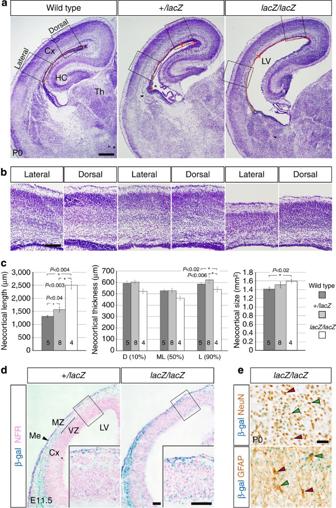Figure 5:Wdfy3lacZ/lacZmice generated through gene targeting exhibit more severe neurodevelopmental defects thanWdfy3disc/discmice. (a) Nissl-stained coronal hemisections through the forebrains of WT, heterozygous and homozygouslacZnewborn pups illustrate the malformations present in affected mutants. The yellow dashed line indicates the cortical length in the WT as measured from the corticostriatal boundary to the ventricular apex. The red dashed line indicates differences in cortical length present in thelacZmutants. (b) Close-ups of cortical segments of lateral and dorsal positions demonstrate cortical thinning inlacZmutants. (c) Bar diagrams showing the results (mean and s.e.m.) of statistical analysis (Student’st-test) for compared morphological parameters. Number (n) of analysed pups and calculatedPvalues of significant changes (asterisks) are indicated in the bar diagrams. Measurements were taken as shown inFig. 1e. (d) Analysis of β-gal expression inWdfy3lacZmice labels Wdfy3+cells and their progeny and confirms at E11.5 dispersed β-gal+cells in the VZ, MZ and meninges (Me). (e) Coronal sections of P0 dorsomedial somatosensory cortex labeled for β-gal expression and immunohistochemically for NeuN and glial fibrillary acidic protein (GFAP) confirms that Wdfy3+progenitors contribute to many neurons and some glia (green arrowheads) but not all NeuN+or GFAP+cells (red arrowheads). Scale bar inais 500 μm, inb200 μm, ind50 μm and ine20 μm. Figure 5: Wdfy3 lacZ/lacZ mice generated through gene targeting exhibit more severe neurodevelopmental defects than Wdfy3 disc/disc mice. ( a ) Nissl-stained coronal hemisections through the forebrains of WT, heterozygous and homozygous lacZ newborn pups illustrate the malformations present in affected mutants. The yellow dashed line indicates the cortical length in the WT as measured from the corticostriatal boundary to the ventricular apex. The red dashed line indicates differences in cortical length present in the lacZ mutants. ( b ) Close-ups of cortical segments of lateral and dorsal positions demonstrate cortical thinning in lacZ mutants. ( c ) Bar diagrams showing the results (mean and s.e.m.) of statistical analysis (Student’s t -test) for compared morphological parameters. Number ( n ) of analysed pups and calculated P values of significant changes (asterisks) are indicated in the bar diagrams. Measurements were taken as shown in Fig. 1e . ( d ) Analysis of β-gal expression in Wdfy3 lacZ mice labels Wdfy3 + cells and their progeny and confirms at E11.5 dispersed β-gal + cells in the VZ, MZ and meninges (Me). ( e ) Coronal sections of P0 dorsomedial somatosensory cortex labeled for β-gal expression and immunohistochemically for NeuN and glial fibrillary acidic protein (GFAP) confirms that Wdfy3 + progenitors contribute to many neurons and some glia (green arrowheads) but not all NeuN + or GFAP + cells (red arrowheads). Scale bar in a is 500 μm, in b 200 μm, in d 50 μm and in e 20 μm. Full size image Wdfy3 lacZ mice express, the lacZ reporter gene, which encodes β-galactosidase (β-gal), a long-lived enzyme that is transferred to the progeny of dividing cells. Consequently, the analysis of β-gal expression allowed us to lineage trace the progeny of Wdfy3 + progenitors. In all stages examined (E11.5, E13.5, E15.5 and P0), the meninges and MZ displayed a high density of β-gal + cells ( Fig. 5d and data not shown). The VZ and SVZ contained β-gal + cells scattered throughout, but often clustered as seen by Wdfy3 immunofluorescence. Occasionally, columns of β-gal + cells could be identified extending radially from the proliferative zones to the cortical plate, which was heavily populated by β-gal + cells at later stages ( Supplementary Fig. 6 ). To confirm the identity of Wdfy3 lineage cells expressing β-gal, we stained sections of P0 brains for β-gal expression and then performed immunohistochemistry to co-label with NeuN, a nuclear marker of mature neurons, and glial fibrillary acidic protein, a cytosolic marker for astrocytes and certain neural progenitors. NeuN staining highly colocalizes with β-gal staining, confirming that many, but not all neurons originate from Wdfy3 + radial glia cells ( Fig. 5e ). Similarly, glial fibrillary acidic protein colocalization is seen for some but not all β-gal + cells demonstrating that Wdfy3 + progenitors also contribute to the astroglial lineage ( Fig. 5e ). The lacZ/lacZ mice exhibit focal cortical dysplasias just as the disc/disc mutants albeit at a higher frequency. The dysplasias typically reach the marginal zone as analysis of both Nissl-stained sections and Tbr1/Ctip2 immunofluorescently labelled sections revealed ( Fig. 6 ). Moreover, the positioning of the observed heterotopias in the lacZ/lacZ mice is not restricted to lateral aspects of the somatosensory area of the neocortex as they are in the disc/disc mice, but can also be found more dorsally in the motor area and can even affect the hippocampus ( Fig. 6b ). In contrast, no focal cortical dysplasias were identified in +/lacZ mice. 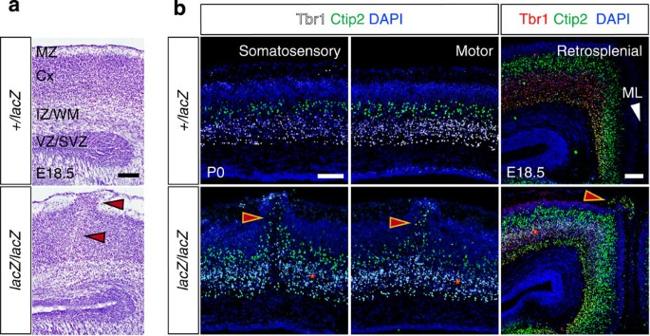Figure 6:Wdfy3lacZ/lacZmice are characterized by widespread focal cortical dysplasias affecting most cortical areas. (a) Nissl-stained coronal sections of the retrosplenial cortex show a focal cortical dysplasia in the homozygouslacZmutant, which disrupts all cortical layers and invades the marginal zone (MZ, arrowheads). (b) Immunofluorescence of cortical lamination markers Tbr1 (layer VI) and Ctip2 (layer V) reveals focal anomalies in the somatosensory and motor cortices of the homozygouslacZmutant at P0 (arrowheads). Asterisks highlight abnormal layer formation through intermingling of Ctip2+neurons with Tbr1+neurons in layer VI. Cx, cerebral cortex; IZ/WM, intermediate zone with white matter; ML midline; MZ, marginal zone; VZ/SVZ ventricular zone/subventricular zone. Scale bars, 100 μm. Figure 6: Wdfy3 lacZ/lacZ mice are characterized by widespread focal cortical dysplasias affecting most cortical areas. ( a ) Nissl-stained coronal sections of the retrosplenial cortex show a focal cortical dysplasia in the homozygous lacZ mutant, which disrupts all cortical layers and invades the marginal zone (MZ, arrowheads). ( b ) Immunofluorescence of cortical lamination markers Tbr1 (layer VI) and Ctip2 (layer V) reveals focal anomalies in the somatosensory and motor cortices of the homozygous lacZ mutant at P0 (arrowheads). Asterisks highlight abnormal layer formation through intermingling of Ctip2 + neurons with Tbr1 + neurons in layer VI. Cx, cerebral cortex; IZ/WM, intermediate zone with white matter; ML midline; MZ, marginal zone; VZ/SVZ ventricular zone/subventricular zone. Scale bars, 100 μm. Full size image To provide a molecular explanation for the observed differences in severity between the disc and lacZ alleles, we sought to examine Wdfy3 protein expression through western blot analysis. We noted that while many Wdfy3 isoforms can be assessed with this method, the largest 400 kDa isoform encoded by full-length Wdfy3 could not be reliably detected, possibly due to a combination of low expression levels, inaccessibility to common lysis protocols and size-dependent inefficient blot transfer. To circumvent this problem, we employed Wdfy3 co-immunoprecipitation to provide for a relative enrichment of Wdfy3 protein in examined lysates. Using this method, we are able to routinely visualize the Wdfy3 400 kDA isoform, but only in WT while in lysates of homozygous disc and lacZ mutants the 400 kDa isoform is always absent ( Supplementary Fig. 7b , full size blots in Supplementary Fig. 9 ). No other isoforms are noticeably affected between mutant genotypes and WT controls. While the observed loss of one Wdfy3 isoform appears plausible for the point mutation of the disc allele, it is somewhat surprising for the lacZ allele, which was generated through homologous recombination involving the insertion of transgenic cassettes carrying stop codons and polyadenylation signals designed to disrupt transcription ( Supplementary Fig. 5 ). To further examine the genetic consequences of the lacZ allele-mediated Wdfy3 gene disruption, we analysed Wdfy3 transcripts through reverse transcription PCR on cDNA samples prepared from E14.5 brains. Using primers that span the transgenic gene disruption, we confirmed alternate read-through transcripts in lacZ allele mutants ( Supplementary Fig. 7c ). In summary, our results provide evidence that both Wdfy3 alleles examined for this study present hypomorphs in which Wdfy3 isoforms are preserved retaining some Wdfy3 function in homozygous mutants of either allele. Two recent studies provided evidence that fragile X mental retardation 1 (Fmr1) protein binds and likely translationally regulates Wdfy3 messenger RNA (mRNA) [7] , [43] . This interesting association prompted us to examine by immunofluorescent analysis whether Fmr1 protein is, possibly through a feedback mechanism, differentially distributed in disc/disc mutants. Analysis, of cortical sections at E15.5 showed no difference in expression levels or distribution of Fmr1 in disc/disc embryos compared with WT ( Supplementary Fig. 8 ). No change in autophagic flux of Wdfy3 disc/disc mutants Previous studies provided evidence that Wdfy3 functions as a scaffolding protein, which directs cargo destined for macroautophagic degradation into autophagosomes. To do so, Wdfy3 directly interacts with the cargo-autophagy receptor complex through P62, the core autophagy machinery through Atg5, and with phosphatidylinositol 3-phosphate of autophagic membranes [20] , [21] , [22] . To gain greater insight into the molecular deregulations caused by loss of Wdfy3 in the disc/disc brain, we next investigated whether there were notable changes in the regulation of macroautophagy, the only cellular process Wdfy3 is currently known to play a role in. To assess macroautophagic flux, we opted to examine protein levels of LC3II and P62, two well-described markers associated with autophagic vesicles [44] , [45] . To that effect, we prepared native forebrain lysates from E12.5 and E15.5 WT and disc/disc mice. Western blot analysis of these lysates showed no significant differences between genotypes when probed with antibodies against LC3 or P62 (Student’s t -test, n =3 for either genotype or stage; Fig. 7a,b ). Furthermore, immunofluorescent analysis in primary neuronal cultures derived from E13.5 WT and disc/disc embryos showed no significant differences in size or density of P62 + puncta (autophagosomes) between the genotypes (Student’s t -test, n =3 for either genotype; Fig. 7c,d ). As Wdfy3 functions as a scaffolding protein for P62-bound ubiquitinated proteins [22] , presumably required for their autophagosomal targeting and subsequent degradation, we examined whether in the disc/disc -mutant brain there is an accumulation of ubiquitinated proteins. Western blot analysis of lysates prepared from E12.5 and E15.5 WT and disc/disc forebrains revealed no significant changes in the total amount of mono- and polyubiquitinated conjugates (Student’s t -test, n =3 for either genotype; Fig. 7e,f ). In summary, our results support the notion that loss of Wdfy3 in the disc/disc mutant does not lead to noticeable changes in autophagic processing during developmental neurogenesis despite the well-characterized role of this molecule in selective macroautophagy. 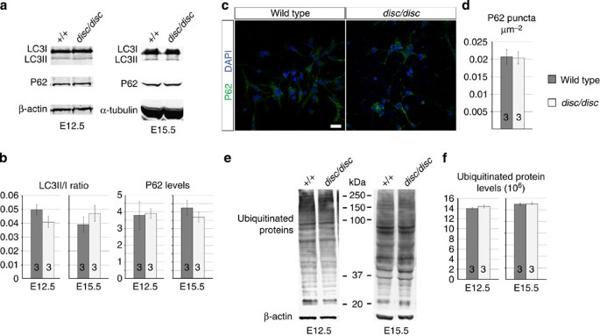Figure 7: No changes in macroautophagic flux ofdisc/discembryos. (a) Western blot analysis of LC3 and P62 on lysates of WT anddisc/disc-mutant brains at developmental stages E12.5 and E15.5 demonstrate no changes in expression levels between the genotypes. (b) Quantification of LC3II/I ratio and P62 levels confirm equal expression levels in the two genotypes. (c) Immunofluorescent analysis of P62 puncta in primary neuronal cultures from WT anddisc/discembryos show no significant differences between the genotypes as quantification results in (d) demonstrate. (e) Western blot analysis of ubiquitinated proteins shows no differences between the genotypes as the quantification of results in (f) demonstrates. All analysis by Student’st-test. Number (n) of samples of either genotype shown in the bar diagrams, which display mean and s.e.m. Scale bar, 20 μm. Figure 7: No changes in macroautophagic flux of disc/disc embryos. ( a ) Western blot analysis of LC3 and P62 on lysates of WT and disc/disc -mutant brains at developmental stages E12.5 and E15.5 demonstrate no changes in expression levels between the genotypes. ( b ) Quantification of LC3II/I ratio and P62 levels confirm equal expression levels in the two genotypes. ( c ) Immunofluorescent analysis of P62 puncta in primary neuronal cultures from WT and disc/disc embryos show no significant differences between the genotypes as quantification results in ( d ) demonstrate. ( e ) Western blot analysis of ubiquitinated proteins shows no differences between the genotypes as the quantification of results in ( f ) demonstrates. All analysis by Student’s t -test. Number ( n ) of samples of either genotype shown in the bar diagrams, which display mean and s.e.m. Scale bar, 20 μm. Full size image Our results demonstrate an essential role for the recently recognized autism factor Wdfy3 in regulating the proliferation of neural progenitors during cerebral cortical neurogenesis in the mouse. Wdfy3 loss-of-function alleles lead to an increase in symmetric proliferative divisions of radial glia, likely at the expense of differentiative mitoses that produce intermediate progenitors. The morphological consequences of this proliferative shift include a longer, thinner and regionally enlarged Cx. Intriguingly, both Wdfy3-deficient mice and a subset of young children on the autism spectrum show abnormal cortical overgrowth in a stereotypical gradient, which is greatest at anterolateral aspects and decreases towards posteromedial areas [26] , [27] , [28] , [29] , [30] . In humans, these anterolateral cortical regions most prone to early overgrowth contain important centres of affective, social and language function suggesting that pathological regional cortical expansion and autism core deficiencies are tightly linked [2] , [12] . A region of particular significance for affective function is the insula of the temporal cortex, an area important for interoception and emotional processing [46] . Social domains important for determining social value, reward and reinforcement include the orbitofrontal cortex, the ventrolateral prefrontal cortex, superior temporal sulcus and the insula [46] , [47] , [48] , [49] , [50] . Repetitive or stereotypical behaviours in autism appear to share characteristics with obsessive–compulsive disorders, which are apparently centred on dysfunctions of the orbitofrontal cortex, further implicating this most anterior cortical domain in the autism pathology [51] . Several cortical and subcortical domains control language function, while expressive language, often impaired in autism, is centred in Broca’s area of the frontal cortex [52] . The importance of frontal cortical aspects in this context was further demonstrated by a recent study, which found that functional connectivity between Broca’s area of the dorsolateral prefrontal cortex to be decreased in autism presenting with language impairments [53] . Importantly, the megalencephaly of affected Wdfy3 mutants presented in this study replicates the gradient of cortical differentiation, which starts anterolaterally and proceeds posteromedially as developmental neurogenesis unfolds [54] . This engrossing correlation suggests that disturbances in the routine of neural progenitor divisions and the associated temporal programme of cortical growth and differentiation may underlie the development of ASDs associated with early brain overgrowth. In particular, an early expansion of the radial glia population through excess symmetric self-renewing divisions leading to an increase in cortical growth may be a crucial component in autism-linked transient megalencephaly. Loss of Wdfy3 provides an explanation for such phenotypic changes by linking defects in progenitor divisions to early brain overgrowth and strongly suggesting an essential role for abnormal proliferation dynamics in the autism pathogenesis. Additional support for the concept of altered neural progenitor divisions in affected Wdfy3 mutants comes from population level analysis of cell cycle progression. In disc/disc mutants the cell cycle is shortened by approximately 30% compared to WT in agreement with the notion that for the cortex to grow larger over the same period of time, progenitor cells will have to divide faster to produce the observed size increase. Several studies have revealed causative links between cell cycle length and mode of progenitor division, with the long-held concept of shorter cycles producing proliferative symmetric divisions [35] , [36] , [37] , [38] being recently challenged by findings that neural progenitors shorten the cell cycle before neurogenic divisions [39] . This latest study seemingly conflicts with the finding of a shortened cell cycle in disc/disc mutants, as the number of Pax6 + radial glia, which are generated exclusively through slower paced, symmetric proliferative divisions, is increased. However, the conflict can be resolved by taking the Tbr2 + intermediate progenitors into account. Intermediate progenitors have a substantially longer cell cycle than radial glia cells [39] and the number of intermediate progenitors in the disc/disc mutants is reduced by about 50%, thus likely overcompensating for the cell cycle length increase of additional radial glia-producing divisions and depressing cell cycle length in our population level analysis. While several studies have identified significant comorbidity of epilepsy with autism, with the co-diagnoses reaching up to 40% of autism cases, the mechanisms underlying this correlation have remained elusive [55] , [56] . A possible explanation for the high prevalence of epilepsy in the autism population is evident from neuropathological studies confirming focal cortical dysplasia, a well-described developmental cause of intractable epilepsy, in children on the autism spectrum [15] , [42] . Additional support for the concept was provided by the analysis of Cntnap2 −/− mice, which show both autism-relevant behavioural deficits and epileptic seizures caused by neuronal migration defects [57] . Our data support these findings by clearly showing that loss of Wdfy3 not only produces an autism-like enlarged cortex but also changes the migratory behaviour of cortical projection neurons resulting in focal cortical dysplasia. Interestingly, we found Wdfy3 message and protein expression to not match exactly in the proliferative compartments of the developing Cx. While Wdfy3 mRNA shows a uniform expression, Wdfy3 protein expression is selectively upregulated in a subset of predominantly dividing progenitors found in the VZ. This unusual finding is not unprecedented, as compared with G-protein signalling modulator 2 (Gsmp2) expression demonstrates. Comparable to Wdfy3, Gsmp2 mRNA expression is present throughout the VZ while Gsmp2 protein is strictly upregulated in dividing progenitors adjacent to the ventricle [58] . While speculative, we suspect that the rapid cycling of radial glia may necessitate the precise timing of transient Wdfy3 upregulation during M phase to be controlled through translation only rather than transcription and translation. This model would suggest that proliferating cells may express Wdfy3 mRNA at all times, awaiting recruitment for translation during mitosis. It is not uncommon to have protein expression tightly regulated at the level of translation, as opposed to regulation at the transcriptional level. Recent analysis of highly sensitive measures of mRNA and protein expression level correlation have shown that mRNA levels only account for up to 40% of the variance of protein abundance levels, with many proteins being expressed from a very small number of message copies [59] . RNA binding proteins, such as Fmr1, are known for their pervasive involvement in translation repression, a tool highly utilized during development to allow for rapid translational activation upon proper signalling within a cell [60] , [61] . While Wdfy3 regulation/activation mechanisms are still not clear, two recent studies have shown that Fmr1 physically associates with Wdfy3 mRNA, which appears supportive of our hypothesis that Wdfy3 expression in dividing neural progenitors is predominantly regulated at the translational rather than the transcriptional level [7] , [43] . Wdfy3 is an unusually large gene of 67 exons in the mouse, a full-length message of approximately 15 kb, and at least nine different predicted splice variants (GenBank Accession numbers XM_006535220.1 — XM_006535228.1 ) Both Wdfy3 alleles analysed in this study appear to be hypomorphs in which several isoforms are preserved while only the largest 400 kDa Wdfy3 isoform is detectably absent in homozygous mutants of either allele. The amino-terminally targeted antibodies (human Wdfy3, residues 500–550) used here to assess protein expression by Wdfy3 co-immunoprecipitation did not show any differences in the isoform profiles between the disc and lacZ allele. Nevertheless, the lacZ allele appears neurodevelopmentally clearly more severely affected than the disc allele, possibly due to the fact that the gene disruption in the lacZ allele occurs earlier (intron 7) than in the disc allele (exon 59), potentially compromising a greater number of splice variants/isoforms not detectable through our means of analysis. Previous studies have characterized Wdfy3 as a component of the macroautophagy pathway, predominantly involved in the selective degradation of specific proteins [20] , [21] , [22] . Consequently, we examined whether loss of Wdfy3 in the brains of disc/disc embryos leads to any overt signs of macroautophagic deregulation. Interestingly, we were unable to detect any differences in autophagic flux between WT and disc/disc mice, as measured by levels of P62 and LC3II expression as well as accrual of ubiquitinated proteins. A possible explanation for this unexpected result may lie in the fact that the disc allele appears to inactivate only the largest 400 kDA Wdfy3 isoform, while other isoforms may still function sufficiently for proper autophagy regulation. Alternatively, Wdfy3 may participate in the selective autophagic targeting of few and low-expressed proteins. As a consequence, neither does the accumulation of these proteins become detectable within the abundance of ubiquitinated proteins nor does it trigger overt changes in autophagy regulation in the disc/disc mutants. Finally, we have to consider that Wdfy3 may fulfil additional functions in the cell other than autophagy regulation and the neurodevelopmental defects of the Wdfy3 mutants are a consequence of autophagy-independent processes. Some support for this notion comes from the fact that no other mutant mouse models with autophagy defects replicate any aspects of the developmental disc/disc pathology. For instance, Ambra1 gt/gt mutants have severe neurodevelopmental anomalies caused by excess proliferation and are exencephalic [62] . In contrast, Snapin −/− -mutant mice have reduced brain size and cell density due to an increase in apoptosis [63] . No neurodevelopmental defects have been reported yet for mutations in genes encoding Atg factors of the core autophagy machinery. Interestingly though, activation of mammalian target of rapamycin, a major regulator of autophagy function leads also to pathological changes in cortical development including the formation of focal cortical dysplasia [64] . Taken together, our study provides seminal evidence that Wdfy3 is a critical regulator of cerebral cortical histogenesis. Loss of Wdfy3 directly affects the proliferation of neural progenitors by shifting the mode of radial glia divisions from differentiative to proliferative. This shift expands the population of radial glia cells, increases cortical size and may be an important component in autism associated with the phenomenon of early brain overgrowth. Positional mapping and candidate gene sequencing The disconnected ( disc ) line was recovered in a forward genetic screen for recessive mutations disrupting forebrain development [23] . Positional mapping was performed by using simple-sequence length polymorphic markers available from the Whitehead Institute for Biomedical Research at MIT. Initial linkage was established after a genome-wide scan with 82 simple sequence repeat markers uniformly spaced across somatic chromosomes on 12 DNA samples from both carriers and affected embryos. For high-resolution meiotic mapping, we scored separate crosses resulting in 131 generated meioses (carriers and embryos counted). Using this approach, we located the disc mutation to an interval on chromosome 5 between markers D5Mit156 (101,537,451–101,537,557 bp) and D5Mit275 (103,997,680–103,997,803 bp) in the NCBI mouse assembly (Build 37.2, current assembly). The identified genetic interval contained 10 protein-coding genes of which all exons were amplified and sequenced from genomic DNA samples. For every set of primers, we used samples of the two parental strains (C57BL/6J and FVB/NJ) and two samples of affected mutants. All primer sequences are available on request. Sequencing of candidate genes was performed at the Ernest Gallo Clinic and Research Center core sequencing facility using Applied Biosystems (Foster City, CA) Big Dye (3.1) reactions. Sequencing reactions were electrophoresed and analysed in an Applied Biosystems Genetic Analyzer 3730XL. Sequence comparisons were carried out using Mutation Surveyor DNA variant analysis software (SoftGenetics, LLC, State College, PA) and BLAST (National Center for Biotechnology Information). Sequences of insufficient quality or read length were dismissed from any comparisons and repeated with revised primer sets. To further confirm that the mutation in Wdfy3 is causative, we genotyped a total of 869 embryos and pups (1,738 meioses) from 108 litters of stages E13.5 to P0, which were easy to score. For genotype analysis, we used a restriction length polymorphism created by the disc allele (additional Dde I site) and confirmed that all 212 affected embryos carried the mutant variant in the homozygous state. The remaining phenotypically WT embryos, were either heterozygous carriers (438) or WT (218) in near perfect Mendelian distribution confirming also the absence of embryonic lethality in mutant embryos. Animal husbandry and genotyping The colony of animals carrying the Wdfy3 disc allele (induced on C57BL/6J background) was maintained by crossing male carriers with FVB/NJ females. This mode of outcross is currently in the fifth generation without any changes in penetrance or variability of the mutant neurodevelopmental phenotype. All embryos presented in the phenotypic analysis of this study were produced from carriers crossed for at least four generations onto an FVB/NJ background. Routine genotyping was performed by amplifying microsatellites D5Mit156 and D5Mit275. Mice were housed in facilities approved by the Association for Assessment and Accreditation of Laboratory Animal Care International. All animals were handled in accordance with protocols approved by the University of California at Davis Institutional Animal Care and Use Committee. Generation of Wdfy3 lacZ and Wdfy3 loxP alleles/colonies The vector construct, targeted embryonic stem cells and chimeric founder mice used for this research project were generated by the trans-NIH Knock-Out Mouse Project (KOMP) and obtained from the KOMP Repository (Project ID: CSD66798; www.komp.org ). The Wdfy3 knockout first, reporter-tagged insertion construct with conditional potential was generated following published protocols [65] . JM8A3.N1 ES cells heterozygous for the Agouti allele [66] were screened for homologous recombination using TaqMan loss-of-negative allele quantitative PCR [67] and the presence of distal loxP cassette. Genomic loss-of-negative allele used the following target primers/probe: forward primer: 5′-AGCCTGGAACTAACAGAAATCCTC-3′, reverse primer: 5′-CCAGTGCAAATAAAGAACTAAATTAGAAGG-3′, probe: 6FAM- 5′-TCTGCCTCTGTACACCACCACA-3′ NFQ. Taqman loxP used the following target primers/probe: forward primer: 5′-GAGATGGCGCAACGCAATT-3′, reverse primer: 5′-TGAACTGATGGCGAGCTCAGA-3′, probe 6FAM—5′-CTTCGTATAGCATACATTATACG-3′—MGBNFQ. Quality control of ES cell clone DEPD00523_5_G11 used for morula aggregation included 5′ arm long-range PCR to reconfirm correct targeting, Taqman quantitative lacZ PCR to confirm single copy integration, confirmation of mycoplasma/parvovirus negative status and chromosome counts of 10 metaphase chromosome spreads. Morula aggregation of targeted ES cells followed published protocols [68] and produced five chimeric founder males ranging from 55–85% ES cell contribution by coat colour assessment. Of these, only one chimera (55% ES coat colour contribution) transmitted the targeted allele to its offspring after breeding to C57BL6/N female mice. The Wdfy3 lacZ line ( Wdfy3 tm1a(KOMP)Mbp ) is maintained as heterozygous mutants on C57BL6/N background. Wdfy3 loxP mice were generated after two successive rounds of breeding of Wdfy3 +/lacZ mice to C57BL/6N- Gt(ROSA)26Sor tm1(FLP1)Dym /Mmucd mice, obtained from the UC Davis Mutant Mouse Regional Resource Center (strain #34413-UCD). Flp/ FRT -mediated recombination produced expected PCR products assessed with Flp primers and absence of lacZ product assessed with lacZ primers ( Supplementary Fig. 4 ). Wdfy3 loxP/loxP mice do not show any overt behavioural or developmental anomalies and are maintained on C57BL6/N background. Oligonucleotide primers used to confirm vector integration ( lacZ primers), correct homologous recombination (5′/3′ arm primers), generation of homozygous mutants from crosses of heterozygote animals (ko primers), and Flp/ FRT -mediated recombination (Flp primers) of the targeted locus are listed below: lacZ left: TTATGGCAGGGTGAAACGCAGGTC, lacZ right: AAACCGACATCGCAGGCTTCTG; 5′ arm external AATGTTTTGAGGTTGAGGGTTAGG, 5′ arm internal TCGGAATAGGAACTTCGGTTCC; 3′ arm internal: AACGCAATTAATGATAACTTCGTATAGC, 3′ arm external: TTGGTCTATCAGACTAAAGACTGG; KO left: ACAGGTCTCTTTGGCTGAGG, KO right: AATGTCTTGCGTCGGAAAAG; Flp forward: AGTGCAAATAAAGAACTAAATTAGAAGG, Flp reverse: CATAACTTCGTATAATGTATGCTATACG. Morphological analysis Comparable 20-μm thick coronal sections of forebrains were Nissl-stained and analysed using Stereo Investigator (MBF Biosciences, Williston, VT). Due to the morphological anomalies of the mutant cortices, thalamic landmarks were used to match sections of different genotypes. Specifically, sections were aligned based on overall thalamic size, shape and extent of the stria medullaris and presence of the anterior thalamic nuclear complex. Neocortical length was measured along the lateral ventricle, from the corticostriatal boundary to the dorsomedial apex as indicated in Fig. 1e . Straight lines extending perpendicularly from the above points to the pial surface defined the neocortical area boundaries, thus taking into account both neocortical thickness and length for area/size assessment. Neocortical thickness was measured at three positions: from the DM apex, measurements were taken at 10% (dorsal (D)), 50% mediolateral (ML) and 90% (lateral (L)) along the total neocortical length, measuring radially from the ventricular surface to the pial surface. RNA in situ hybridization RNA in situ hybridization was performed on 20-μm thick sections of cryopreserved tissue from fixed E14.5 embryos using standard methods previously described [69] . Digoxigenin-labelled Wdfy3 riboprobes were generated from an 864 bp cDNA fragment (nucleotides 4,429–5,292 of NM_172882) ligated into the TOPO TA PCR4 vector (Invitrogen, Life Technologies, Grand Island, New York). In vitro transcription was performed on linearized plasmids isolated from bacterial clones to produce DIG-labelled anti-sense (linearized with Not I, transcribed with T3 RNA polymerase) and sense probes (linearized with Spe I, transcribed with T7 RNA polymerase). RNA in situ hybridization experiments as well as all other histological analyses were performed at least three times on at least three embryos of each genotype and representative results documented. Immunofluorescence and EdU labelling Depending on developmental stage, embryos were fixed by immersion (up to E13.5) or perfusion in 4% paraformaldehyde (PFA) in phosphate-buffered saline (PBS). Subsequently, tissue was fixed for an additional 1–2 h, immersed in 15% and then 30% sucrose in PBS, and cryoprotectively frozen to be sectioned at 8–20 μm. Immunofluorescence was carried out on slide-mounted sections according to standard protocols using the following primary antibodies: mouse α-Wdfy3, 1:250 (Abnova, Taiwan); rabbit α-Pax6, 1:200 (Covance, Dedham, MA); rabbit α-Tbr2 1:400 (Abcam, Cambridge, MA); rabbit α-Histone H3 1:500 (Abcam, Cambridge, MA). After labelling procedures tissue sections were postfixed in 4% PFA in PBS and mounted with Fluoromount-G (Southern Biotech, Birmingham, AL). For the 24 h EdU pulse-chase assay, time-pregnant females were injected intraperitoneally with 50 mg kg −1 bodyweight EdU. After 24 h, females were killed, and embryo tissue processed as described above. Slides were incubated in 2N HCl at 37 °C for 20 min and rinsed two times in PBS with 0.2% Triton X-100. EdU detection was performed after immunostaining according to manufactures Click-it EdU Alexa 594 imaging kit protocol (Life Technologies, Carlsbad, CA). The fraction of cells that had exited the cell cycle (Q-fraction) was estimated by counting the numbers of BrdU + /Ki67 − cells basal to the SVZ and all BrdU + cells in 200 μm cortical segments. Q-fractions were calculated by dividing the number of BrdU + /Ki67 − cells by the total number of BrdU + cells. All imaging was carried out on a Nikon Eclipse C1 laser scanning confocal microscope with D-Eclipse C1 si camera. Single- and merge-channel views were acquired with the associated Nikon EZ-C1 3.90 FreeViewer software. All quantifications of labelled cells were carried out at equivalent positions on 3–4 sections of every brain and averaged for every sample. Analysis of cell cycle kinetics To assess cell cycle progression a dual thymidine labelling approach was used. EdU was administered through intraperitoneal injection to time-pregnant females at 50 mg kg −1 followed by BrdU injection at 50 mg kg −1 1.5 h later. Litters of 13.5-day-old embryos were collected 30 min after the BrdU injection, fixed in 4% PFA in PBS, brains frozen in 30% sucrose in PBS and coronally cut at 12 μm on a cryomicrotome. Slides were incubated in 2 N HCl at 37 °C for 20 min and rinsed in PBS with 0.2% Triton X-100 before immunostaining with α-BrdU monoclonal antibodies (1:10; Life Technologies), α-Ki67 antibodies (1:200, Abcam, Cambridge, MA), and Click-iT EdU detection following the manufactures instructions (Life Technologies). Subsequently, mediolateral cortical aspects were imaged as described above and labelled cells of 200 μm wide cortical segments counted. Calculation of cell cycle parameters followed established paradigms [40] , [41] . Specifically, the duration of the experiment ( T I ) was divided by ratios of single (EdU + ) over double-labelled cells (EdU + /BrdU + ) to generate estimates of S-phase length ( T S ). To estimate total cell cycle length ( T C ), T S was divided by the ratio of EdU + /BrdU + cells over Ki67 + cells. X-gal staining Staining for β-gal activity expressed by the lacZ reporter of the targeted Wdfy3 allele was performed using X-gal as a substrate on 20 μm coronal forebrain cryosections according to standard protocols as previously described [23] . Western blot analysis A quantity of 75 μg of protein per well were loaded into NuPAGE 12% Bis-Tris gels (Life Technologies). After electrophoresis and transfer to PVDF membranes, Odyssey blocking buffer was applied (Li-Cor, Lincoln, NE) for 1 h at room temperature. Subsequently, membranes were incubated overnight at 4 °C with the following primary antibodies diluted in Odyssey blocking buffer including 0.1% Tween-20 and 0.05% NaN 3 : α-P62 (1:1,000; Progen, Heidelberg, Germany), α-LC3 (1:250; Novus, Littleton, CO) and α-multiubiquitin (1:1,000; Enzo, Farmingdale, NY). Secondary antibodies were applied for 1 h at room temperature (Li-Cor α-rabbit, 1:10,000; Li-Cor α-guinea pig: 1:5,000). The PVDF membrane was then imaged on the Li-Cor Odyssey imaging system and quantified using the Li-Cor image studio software. Following the initial probing and analysis, the membrane was blotted with antibodies against β-actin (1:8,000; Proteintech, Chicago, IL) or α-tubulin (1:2,500; Sigma, St Louis, MO) as loading controls. Wdfy3 co-immunoprecipitation Whole E13.5 embryos were lysed in lysis buffer consisting of 50 mM Tris–HCl pH 7.4, 150 mM NaCl, 1 mM EDTA, 1% Triton X-100, supplemented with protease inhibitor cocktail tablet (Roche, Indianapolis, IN). Lysates containing 1 mg of protein were incubated with α-Wdfy3 antibody (Novus) overnight and then immunoprecipitated using Dynabeads Protein A Immunoprecipitation Kit (Life Technologies). Subsequently, total protein lysates, immunoprecipitated and flow-through samples were electrophoresed in NuPAGE 3–8% Tris-Acetate gels (Invitrogen, Carlsbad, CA). Proteins were transferred to PVDF membranes and blocked in Odyssey blocking buffer (Li-Cor Biosciences). Membranes were incubated with α-Wdfy3primary antibody (1:1,000; Novus) diluted in Odyssey blocking buffer containing 0.1% Tween-20, overnight at 4 °C, washed with 0.1% Tween-20 in PBS, before incubating with Li-Cor IR secondary antibody (1:5,000; Li-Cor Biosciences) in Odyssey blocking buffer washed, and imaged on the Li-Cor Odyssey IR scanner. The 333 kDA Wdfy3 isoform, present in all samples served as loading control. Reverse transcription PCR Total RNA was purified from E14.5 embryos using the RNAeasy Mini Kit (Qiagen, Germantown, MD). cDNA was generated form 5 μg total RNA using Omniscript RT kits (Qiagen) following the manufacturers’ directions. PCR was conducted using the following primers: RT forward: 5′-TCCTGCCAGTGTTTAACAGG-3′, RT reverse: 5′-ATCCGAAAATCATCCAGCAG-3′. Primary neuronal cultures and P62 puncta counts Primary neurons were obtained and cultured from E12.5 brains of WT and disc/disc mice following standard protocols [70] . In brief, following euthanasia embryos were removed from the uterus of timed pregnant females. After dissecting the brain from the skull, it was placed in ice-cold PBS, the forebrain cut into 1 mm sized cubes and treated with 0.25% Trypsin–EDTA for 10 min at 37 °C. Subsequently, neurobasal medium with B27 supplement was added, the tissue dissociated through repeated pipetting and passed through a 70 μm nylon strainer to obtain single-cell suspensions. The suspensions were added dropwise to poly- D -lysine-coated 12 mm round coverslips (BD Biosciences, Franklin Lakes, NJ) and allowed to grow at 37 °C in a humidified CO 2 incubator until the cells reached ~50–70% confluence. For immunocytochemistry, cells were briefly fixed in 4% PFA in PBS, blocked and permeabilized (10% donkey serum, 1% Triton X-100 in PBS) for 1 h, before being incubated overnight with P62 polyclonal antibody (1:125; Progen). After for 1 h of secondary antibody incubation with Alexa Fluor 488 Donkey α-mouse (1:1,000; Molecular Probes, Eugene, OR), cells were counterstained with 4′,6-diamidino-2-phenylindole. Slide-mounted coverslips were imaged with an Olympus C-1 inverted confocal microscope and Stereo Investigator digital imaging software, version 10.21.1. Eight to ten unbiased images of each cover slip were taken by imaging first the outer rim of the cover slip, and then taking each picture thereafter by rotating the disc ~90° from the previous position. After the first four pictures were taken, the next set of four was taken closer to the centre of the cover slip. To count P62 puncta, a standard was set up that defined each punctum as having three adjacent pixels with a qualitatively bright net intensity. As cell size can vary considerably and number of puncta correlates with cell size, we decided to calculate the number of puncta as a ratio over visible cell surface in μm 2 . Consequently, cells were only analysed when nuclei were clearly visible and the cell outline was discernible within the plane of focus. P62 puncta counters were blinded to genotypes and trained on the same pictures to ensure comparability. Puncta μm −2 were then summed and divided by the number of cells in the corresponding genotype. Averages and s.d. values of puncta counts were calculated and the two genotypes were compared side-by-side. How to cite this article : Orosco, L. A. et al. Loss of Wdfy3 in mice alters cerebral cortical neurogenesis reflecting aspects of the autism pathology. Nat. Commun. 5:4692 doi: 10.1038/ncomms5692 (2014).